Fish parasites resolve the paradox of missing coextinctions Models of coextinction identify parasites as one of the most menaced ecological groups. The number of host species a parasite uses should strongly affect its risk of coextinction. The naïve expectation is that the lower the number, the higher is the parasite’s risk of being left with no hosts. Here we analyse the coextinction risk of 12,141 fish parasite species and find that highly specific parasites are not the most endangered, because they tend to use hosts with low vulnerability to extinction. This unexpected result may explain why the number of documented host–parasite coextinctions is much lower than predicted by theoretical studies. Coextinction, that is, loss of a species as a result of extinction or local extirpation of an associated species, is thought to have an important role in accelerating the global biodiversity decline [1] , [2] . However, coextinctions seem surprisingly less common than expected [3] , [4] . Specialization is one of the main factors affecting species extinction risk [5] , for both free living organisms and symbionts [4] . Many parasite species have very restricted host relationships, and hence are thought to be at great risk to become extinct together with their hosts [6] . Thus, it is reasonable to estimate the probability of a parasite species to go coextinct on the basis of its specificity and of the vulnerability of its hosts [2] , [6] . However, little is known about the potential relationships between the number of hosts a parasite uses, and the vulnerability of these hosts. In the present paper, we investigate this issue using a large data set (FishPEST) of fish parasites. We computed the extinction risk of 12,141 fish parasite species belonging to the major helminth groups (Acanthocephala: 581 species; Cestoda: 1,520 species; Monogenea: 4,325 species; Nematoda: 1,468 species; Trematoda: 4,247 species) as the product of the extinction probabilities of their respective known fish host species. In addition, for each parasite species, we calculated the average vulnerability of their fish hosts. We did not make any distinction among the possible different roles played by different fish hosts in parasite life cycles, as the vulnerability of intermediate and definitive host species contributes equally to the overall endangerment of a parasite species [4] . However, we recognize that our database might be affected by various biases, and particularly: (1) the fact that we did not consider possible non-fish intermediate hosts may lead to an underestimation of host ranges; (2) we considered all hosts as equally exploited by parasite species, which may inflate the contribution to parasite extinction risk by hosts that are rarely used; (3) some fish species might be over-sampled (for example, fish with commercial value whose parasites are well known) and others might be under-sampled (for example, rare fish scarcely examined for parasites); (4) host–parasite relationships are not equally well known at a global scale. To assess the potential effects of these biases on our general results, we constructed and analysed separately four reduced host–parasite data sets (see Methods for details) including: (1) only parasite species that use exclusively fish species as hosts; (2) only frequently observed parasite–host pairs; (3) only well-sampled parasites (for example, occurring on at least 10 hosts); and (4) only Nearctic records, being the Nearctic fish fauna the most sampled one in the used databases. We find that, contrary to expectation, in all analysed data sets, the most specialized parasites are not the most endangered ones, because they tend to be associated with fish species that have low vulnerability. Thus, specialized parasites use few, but less vulnerable hosts, which reduces coextinction risk. This evolutionary strategy may explain why highly specialized parasites are not so prone to extinction. Parasite specificity and host vulnerability Using the full FishPEST data set, we found that Monogenea were the most specialized parasites, with a mean host range lower than those of any other parasite group ( Fig. 1a ). This should imply a higher extinction risk [1] , but we found that the average risk of extinction of Monogenea was lower than those of less specialized parasite groups, such as Cestoda and Nematoda ( Fig. 1b ). We also found that Monogenea were the parasites that occurred, on average, on the least vulnerable hosts ( Fig. 1c ). Thus, for these parasites, the endangerment due to the narrow range of their hosts is counterbalanced by the fact that such hosts are among the less vulnerable. Use of reduced data set gave similar results ( Supplementary Fig. S1 ): in all the analyses, the Monogenea had always the smallest host range and the lowest average host range vulnerability, but never had the highest extinction risk. 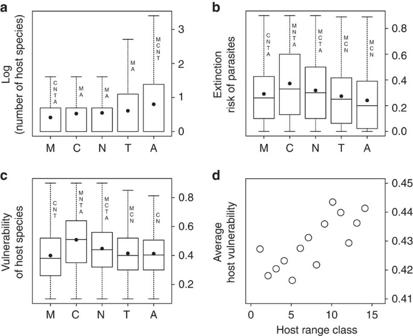Figure 1: Relationships between parasite specificity and host vulnerability. (a) Parasite–host range; (b) parasite coextinction risk; (c) vulnerability of host fish. Boxes indicate first and third quartiles, whiskers indicate range values, black dots within boxes indicate mean values, and horizontal lines indicate median values. Letters alongside whiskers indicate the parasite groups whose corresponding values significantly differ (P<0.05) from that of the group under examination. (d) Relationship between mean vulnerability of the hosts of each class and host range classes (Spearman rank correlation coefficientrs=0.7,P<0.0001); thexaxis is a geometric series with common ratio of 1.5 (minimum value=1; maximum value=292). Parasite groups: A: Acanthocephala, C: Cestoda, M: Monogenea, N: Nematoda, T: Trematoda. Figure 1: Relationships between parasite specificity and host vulnerability. ( a ) Parasite–host range; ( b ) parasite coextinction risk; ( c ) vulnerability of host fish. Boxes indicate first and third quartiles, whiskers indicate range values, black dots within boxes indicate mean values, and horizontal lines indicate median values. Letters alongside whiskers indicate the parasite groups whose corresponding values significantly differ ( P <0.05) from that of the group under examination. ( d ) Relationship between mean vulnerability of the hosts of each class and host range classes (Spearman rank correlation coefficient r s =0.7, P <0.0001); the x axis is a geometric series with common ratio of 1.5 (minimum value=1; maximum value=292). Parasite groups: A: Acanthocephala, C: Cestoda, M: Monogenea, N: Nematoda, T: Trematoda. Full size image Predictors of extinction risks A multivariate analysis of variance revealed that parasite groups differed for parasite extinction risk, number of known hosts and vulnerability of their hosts (Wilks’ λ =0.947, F=55.2, P <0.001; see also Supplementary Table S1 ). When the overall data set was analysed, post-hoc comparisons (with Bonferroni corrections) revealed significant ( P <0.001) pairwise differences in parasite extinction risk for all groups except between Acanthocephala and Trematoda. Parasites also differed ( P <0.001) in the vulnerability of their hosts (except for comparisons of Acanthocephala with Trematoda and Monogenea) and host range (except for comparisons of Nematoda with Trematoda and Cestoda, and of Trematoda with Cestoda). An analysis conducted with only frequently used hosts ( Supplementary Fig. S1-IV ) gave virtually identical results in post-hoc pairwise comparisons. By contrast, when the analysis was restricted to parasites that only use fish hosts ( Supplementary Fig. S1-I ), post-hoc comparisons revealed insignificant ( P >0.05) pairwise differences in parasite extinction risk for all comparisons involving Acanthocephala, for Nematoda versus Cestoda, and for Trematoda versus Monogenea. In this data set, parasites also differed ( P <0.001) in the vulnerability of their hosts (except for comparisons of Acanthocephala with Trematoda and Monogenea, and of Trematoda with Monogenea) and host range (except for comparisons of Nematoda with Trematoda and Cestoda, and of Trematoda with Cestoda), in accordance with the results of the most comprehensive analysis. When only parasites with more than 10 hosts were considered, post-hoc tests revealed no significant differences in pairwise comparisons for parasite extinction risk, but significant ( P <0.01) differences occurred for host vulnerability in all comparisons (except in those involving Acanthocephala, which were significantly different only from Nematoda at P <0.05). In this analysis, parasites also differed ( P <0.001) in their host range in all pairwise comparisons, except for comparisons of Nematoda with Trematoda and Cestoda, and of Trematoda with Cestoda, in accordance with previous analyses. Use of only Nearctic parasites–hosts produced very similar results: post-hoc tests revealed no significant differences in pairwise comparisons for parasite extinction risk, but indicated significant ( P <0.01) differences for host vulnerability in all comparisons (except those involving Nematoda and Acanthocephala, which were significantly different only from Monogenea at P <0.05). In this analysis, parasites also differed ( P <0.001) in their host range in all pairwise comparisons, except in comparisons of Nematoda with Trematoda and Cestoda, and of Trematoda with Cestoda, in accordance with previous analyses. Parasite extinction risk corrected for host traits An analysis of covariance ( Table 1 and Supplementary Table S2 ) showed that when the effects of host vulnerability and host range were used as covariates, parasites differed ( P <0.05) in their extinction risk in all pairwise comparisons for the overall data set, in all pairwise comparisons except the couple Monogenea versus Nematoda when only parasites with more than 10 hosts were considered, and in all comparisons except the couples Nematoda versus Cestoda and Trematoda versus Monogena when only parasites using fish hosts were analysed. No pairwise significant difference was found for the data sets including only the Nearctic species and only the species with more than 10 hosts. Table 1 Results of analysis of covariance for extinction risk of helminth parasites of fish. Full size table After removing all differences that can be accounted for by the covariates (host vulnerability and host range), least squares means (that is, the expected population marginal means, given the current model) indicated Monogenea as a group with a high extinction risk ( Fig. 2 ; analyses conducted using the reduced data sets produced analogous patterns). This confirms that the low extinction risk exhibited by Monogenea is the result of the low vulnerability of their hosts. 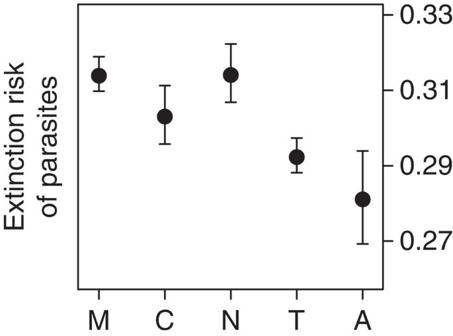Figure 2: Parasite extinction risk. Least squares means of parasite extinction risk after analysis of covariance (ANCOVA) with host vulnerability and host range used as covariates. Vertical bars denote 95% confidence intervals. Parasite groups: A: Acanthocephala, C: Cestoda, M: Monogenea, N: Nematoda, T: Trematoda. Figure 2: Parasite extinction risk. Least squares means of parasite extinction risk after analysis of covariance (ANCOVA) with host vulnerability and host range used as covariates. Vertical bars denote 95% confidence intervals. Parasite groups: A: Acanthocephala, C: Cestoda, M: Monogenea, N: Nematoda, T: Trematoda. Full size image Nestedness analysis Using the complete data set, we also compiled a presence/absence matrix of all parasite species (rows) per all host species (columns) to test host–parasite network nestedness (see Fig. 3 ). This matrix resulted significantly nested (Brualdy and Sanderson discrepancy, Z =−9.61, P <0.001). 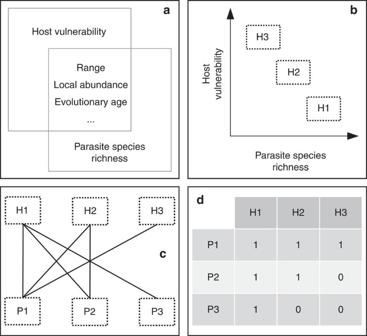Figure 3: Basic characteristics of host–parasite networks. Schematic representation of the theoretical linkages between the determinants of host vulnerability, parasite species richness per host, and nestedness in host–parasite networks. Some of the characteristics of a host (such as its distribution range, local abundance, evolutionary age, etc.) that affect its vulnerability may also influence the number of parasite species using that host (a). Thus we may expect to find more parasites in low vulnerable hosts (for example, host H3) than in high vulnerable ones (for example, host H1) (b). In host–parasite networks, specific parasite species (P1, P2, P3) are mainly linked to hosts characterized by high parasite species richness (c). This is consistent with both the commonness of nestedness patterns in host parasite networks (d) and with our results, providing an indirect support to the hypothesis that highly specific parasites may reduce their coextinction risk by predominantly using low vulnerable hosts. Figure 3: Basic characteristics of host–parasite networks. Schematic representation of the theoretical linkages between the determinants of host vulnerability, parasite species richness per host, and nestedness in host–parasite networks. Some of the characteristics of a host (such as its distribution range, local abundance, evolutionary age, etc.) that affect its vulnerability may also influence the number of parasite species using that host ( a ). Thus we may expect to find more parasites in low vulnerable hosts (for example, host H3) than in high vulnerable ones (for example, host H1) ( b ). In host–parasite networks, specific parasite species (P1, P2, P3) are mainly linked to hosts characterized by high parasite species richness ( c ). This is consistent with both the commonness of nestedness patterns in host parasite networks ( d ) and with our results, providing an indirect support to the hypothesis that highly specific parasites may reduce their coextinction risk by predominantly using low vulnerable hosts. Full size image In contrast with the common assumption that Monogenea are the most menaced group of parasites as a consequence of their host specificity [1] , we found that these parasites are not the most threatened, because they tend to use hosts with low vulnerability to extinction. These findings have important implications. From an evolutionary perspective, highly specific parasites, such as the Monogenea, would be expected to evolve stable relationships mostly with host species that are easily encountered and infected, as indicated by the ubiquity of nestedness in antagonistic networks [7] . In a nested host–parasite network (such as that used in this study), generalist parasites are present on most host species, whereas specific parasites are mainly present on host species with high parasite species richness (see Fig. 3d ). Some features of a host that increase the number of parasite species occurring on it may also be directly or indirectly related to host vulnerability. For example, hosts having a wide distribution and a high local abundance (that are features significantly intercorrelated in both freshwater and marine fish [8] ) are likely to bear many parasite species [9] , [10] and, at the same time, to be less endangered than rare species [11] . Thus, some species-level host traits that increase nestedness of host–parasite networks could also reduce the coextinction risk of highly specific parasites by favoring their distribution towards less vulnerable hosts (see Fig. 3 ). For parasites of fish, we found that average host vulnerability tends to be higher in those fish species that are used by more generalist parasite species ( Fig. 1d ), whereas highly specialized parasite species tend to infect fish species with low vulnerability. This relationship between parasite specialization and host vulnerability, which is consistent with the important role in biodiversity conservation attributed to nestedness of facilitative networks [12] , [13] , [14] , suggests a general solution to the paradox of missing host–parasite coextinctions. Host vulnerability and parasite extinction risk We obtained host–parasite records ( n =38,567) and vulnerability values of host species ( n =4,682), respectively, from FishPEST [15] , [16] ( http://purl.oclc.org/fishpest ) and FishBase [17] ( www.fishbase.org ). FishBase computes vulnerability values using a fuzzy expert system integrating biological and ecological characteristics of fish species [18] . These values of host vulnerability range from 0 (minimum vulnerability) to 100 (maximum vulnerability). We used these values (divided by 100) as measures of the probabilities of host species to go extinct. The extinction risk of a parasite species depends on how many host species it uses and on the vulnerability of these host species, with parasites occurring on more hosts expected to be less prone to extinction. Thus, for each parasite, we calculated the extinction risk as the product of the extinction probabilities of its known host species (for example, if host A has 0.1 probability of going extinct, and host B has 0.1 probability of going extinct, then a parasite associated with hosts A and B has a probability 0.1 × 0.1=0.01 of going extinct). Also, for each parasite, we calculated the average vulnerability of their hosts, as the arithmetic mean of the vulnerability values (divided by 100) of their known hosts, and its host range (that is, the number of known hosts). Statistical analyses We used a multivariate analysis of variance to test if parasite groups differed for parasite extinction risk, number of known hosts and vulnerability of their hosts. We applied an analysis of covariance to test for differences in extinction risk among parasite groups using host vulnerability and host range as covariates. Then we used Bonferroni procedures to adjust significance levels in post-hoc comparisons. We developed our main analyses omitting intermediate hosts different from fishes although it is well known that many parasites use other hosts, for example, invertebrate species. Including intermediate hosts might be useful to take into account the role of non-fish hosts in the coextinction process. For example, a parasite with several fish hosts may have a single intermediate non-fish host that may act as a key coextinction driver; not considering this intermediate host may produce an underestimation of the risk of coextinction. However, data about intermediate hosts different from fish are very scarce, especially for the invertebrates. Many invertebrates (for example, mollusks and crustaceans) are reported as intermediate hosts for many parasites, but they are very rarely identified to species level, which makes it impossible to introduce them in the calculation of host range. Moreover, for most non-fish hosts (and especially for invertebrates), calculating extinction risk may not be possible, or at least not with the same rigorous criteria used to compute vulnerability of fish species [18] . Thus, to assess if patterns depicted by our general analyses might be biased by omitting non-fish hosts, we performed analogous analyses using a subset of parasite species only associated with fish species. For this, we made use of the databases of the Natural History Museum (London) [19] and of the US parasitological collection [20] , which are the main data sources of FishPEST database. From these databases, we excluded all helminth species known to use hosts different from fish. This way, we constructed a reduced data set including 24,651 records of helminth species that use exclusively fish hosts. This ensures that the analyses conducted using this reduced data set are not biased by the risk of extinction of unconsidered intermediate hosts different from fish. A second problem is due to the fact that our computation of parasite extinction risk is based on the assumption that all host species are equally exploited by their known parasite species, which is clearly an approximation of ecological reality. To assess if this may bias our conclusions, we created a data set by taking into account all the fish parasite records included in the Natural History Museum database and by excluding, for each parasite species, all the poorly exploited hosts. To do that we counted the number of records (that is, literature citations) for each host–parasite couple. Then, for each parasite species we considered only the hosts that have been reported in association with the parasite a number of times not smaller than half that of the host species most frequently associated with the parasite species (that is, for each host record we adopted a threshold computed as n/n max ≥0.5, where n is the number of times the host species under examination has been reported in literature from the considered parasite species, and n max is the n value of the host species most reported from the considered parasite species). This way, we restricted the analyses to fish species that cannot represent occasional hosts, but that are important hosts for a given parasite species. Host species more frequently investigated (for example because of their commercial value) may appear to be used by more parasite species than less investigated hosts. Many fish species have been examined at very few locations and/or for a limited subset of parasite taxa [21] . To take into account this possible bias, we reduced the FishPEST database by excluding fish species known to harbour <10 parasite species. Similarly, because of possible differences in sampling efforts among regions, we performed the same analyses using a subset of FishPEST data including only Nearctic parasites, which are those most investigated in respect to the ratio between sampled hosts and known hosts for the biogeographic region ( ∼ 40% according to FishBase). For the complete data set, we also tested if vulnerability of the hosts was correlated with the host range of the parasites. For this, we divided parasite species into 14 classes according to their host range size. We defined these classes using a geometric series to couple with the pronounced skewness of parasite–host range towards low values (see Supplementary Fig. S2 ). We used a common ratio of 1.5 as a tradeoff between number of intervals and number of parasite species per interval. Table 2 reports the lower and upper limits of each class (that is, the minimum and maximum number of hosts used by a parasite) and the number of parasite species per class. Then for each class we calculated the average vulnerability of the hosts used by all parasite species falling in that class of host range. Finally, we used a Spearman rank coefficient to correlate host range classes with average vulnerability. Table 2 Host range classes. Full size table Nestedness analysis We used the complete data set to compile a presence/absence matrix of parasites species (rows) per host species (columns). Then we measured nestedness of this matrix using the Brualdi and Sanderson discrepancy index (BR) [22] . To evaluate the significance of the BR index, we created 100 null matrices of the same size of the original matrix (12,141 rows × 4,682 columns), attributing to each cell a probability of being occupied equal to the average of the probabilities of occupancy of its row and column, in order to take into account both parasite–host specificity and parasite species richness per host species [23] . Finally, we computed a Z- value as the difference between BR index of the original matrix and the mean value of the BR indexes of the null matrices, quoted by the standard deviation of the BR indexes of the null matrices [22] . We performed all nestedness analyses using the software NeD ( http://ecosoft.alwaysdata.net ), which has no limitations on matrix size. How to cite this article: Strona, G. et al . Fish parasites resolve the paradox of missing coextinctions. Nat. Commun. 4:1718 doi: 10.1038/ncomms2723 (2013).